Interpolar microtubules are dispensable in fission yeast meiosis II The mitotic spindle consists of two types of microtubules. Dynamic kinetochore microtubules capture kinetochores, whereas stable interpolar microtubules serve as the structural backbone that connects the two spindle poles. Both have been believed to be indispensable for cell division in eukaryotes. Here we demonstrate that interpolar microtubules are dispensable for the second division of meiosis in fission yeast. Even when interpolar microtubules are disrupted by a microtubule-depolymerizing drug, spindle poles separate and chromosomes segregate poleward in second division of meiosis in most zygotes, producing viable spores. The forespore membrane, which encapsulates the nucleus in second division of meiosis and is guided by septins and the leading-edge proteins, is responsible for carrying out meiotic events in the absence of interpolar microtubules. Furthermore, during physiological second division of meiosis without microtubule perturbation, the forespore membrane assembly contributes structurally to spindle pole separation and nuclear division, generating sufficient force for spindle pole separation and subsequent events independently of interpolar microtubules. Microtubules have essential functions in cell division of eukaryotes. The mitotic spindle consists of two types of microtubules: kinetochore microtubules (ktMTs) and interpolar microtubules (ipMTs) [1] , [2] , [3] . ktMTs dynamically repeat polymerization and depolymerization of α/β-tubulin dimers, thereby capturing and pulling kinetochores of chromosomes. By contrast, stable ipMTs serve as the structural backbone connecting the two spindle poles [4] . The necessity of spindle microtubules for chromosome segregation has been demonstrated in many studies for the last few decades, using drug or cold treatment to depolymerize microtubules, as well as using mutant cells defective in microtubule organization. The requirement of ktMTs appears evident, as a failure in kinetochore-microtubule attachment can cause aneuploidy [5] . The microtubule-associated protein Ase1/PRC1 is known to bundle ipMTs at the spindle midzone in late mitosis (anaphase) [6] , [7] , [8] , [9] . Dysfunction of Ase1/PRC1 does not affect kinetochore microtubule attachment in metaphase, but causes a spindle collapse in anaphase, which frequently leads to production of aneuploids. Aneuploidy can drive genomic instability and is therefore closely related to tumourigenesis [10] . Thus, both types of microtubules are believed to be indispensable for proper chromosome segregation in eukaryotes. Most of this knowledge, however, is based on studies of mitotic cells, and whether this property is shared with meiotic cells is poorly understood. In this study, we performed live-cell observations in both mitotic and meiotic cells of the fission yeast Schizosaccharomyces pombe to re-evaluate the biological significance of microtubules in chromosome segregation. We added a microtubule-depolymerizing drug, methyl-2-benzimidazole-carbamate (MBC), to wild-type cells before mitotic or meiotic division and monitored the cell-cycle progression using real-time fluorescence microscopy ( Supplementary Fig. S1a for the S. pombe lifecycle). We found that ipMTs are dispensable in second division of meiosis (MII), against the general belief of an absolute requirement of the microtubules. Spindle pole separation and subsequent events occurred normally even in the absence of ipMTs in MII. Furthermore, we identified that the forespore membrane, which encapsulates the nucleus, is responsible for generation of the force to separate the poles instead of microtubules. Unexpectedly, even when microtubules were intact, removal of the forespore membrane reduced the ratio of spindle pole separation. We propose that the forespore membrane is the first non-microtubular material that produces the force for cell division under physiological conditions. Interpolar microtubules are dispensable in MII Microtubules were visualized with green fluorescent protein (GFP)-tagged α2-tubulin (Atb2), the spindle pole body (SPB; a fungal centrosome equivalent) was labelled with the cyan fluorescent protein (CFP)-tagged SPB half-bridge component Sfi1 (Sfi1-CFP) and kinetochores were labelled with 2mCherry-tagged Mis6 (Mis6-2mCh). During normal mitosis in the absence of MBC, microtubules that were nucleated from the two SPBs interacted to form a robust bipolar spindle and separate the SPBs [11] , [12] ( Fig. 1a ). Until metaphase, the central region of the spindle exhibited a relatively dim GFP-Atb2 signal (12 min), reflecting the fact that a number of short ktMTs were located near the SPBs, whereas ipMTs were connecting the two SPBs [4] ( Supplementary Fig. S1b for a schematic). In anaphase B (22 min), the spindle elongated through the sliding of interdigitating ipMTs at the spindle midzone. Similar properties were observed for the spindle in meiosis I (MI) and in MII ( Fig. 1b , Supplementary Fig. S1c ). We added MBC and observed cells that had just entered mitosis. As expected, microtubule nucleation from SPBs was severely inhibited, and SPBs never separated in the presence of MBC (90 min; Fig. 1c and Supplementary Fig. S1d ), confirming the significance of microtubules in mitotic division. In contrast, when MBC was added to zygotes before MII (0 min; Fig. 1d ), SPBs could separate, even though microtubule nucleation was considerably inhibited by MBC ( Supplementary Fig. S1e ). A GFP-Atb2 signal was detected only around the spindle poles, indicating that ipMTs connecting the two SPBs were disrupted (42 min). In the presence of MBC, only short microtubules associated with kinetochores were detected ( Fig. 1e ), suggesting that they might serve as ktMTs. Kinetochores separated equally to the two poles in most MBC-treated cells (see below), indicating that the short microtubules were sufficient for the capture and connection of kinetochores to the SPBs. Not only SPB separation and chromosome segregation but also nuclear division was carried out successfully in the presence of MBC ( Fig. 1f ). 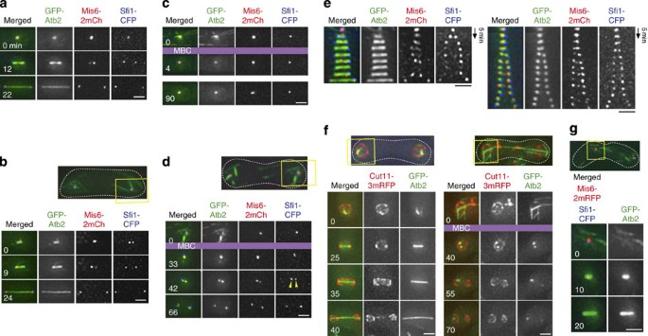Figure 1: SPB separation with chromosome segregation and nuclear division occurred without interpolar microtubules (ipMTs) in meiosis II. (a–e) Live-cell imaging of cells carrying GFP-Atb2 (microtubules; green), Mis6-2mCherry (Mis6-2mCh; kinetochores; red) and Sfi1-CFP (SPBs; blue). Time-lapse images of cells undergoing normal mitosis (a) and meiosis II (MII) (b) are shown. For MII cells inbandd, the boxed regions of zygotes are shown enlarged as time-lapse images. The shape of cells is outlined in dotted curves;n=10. (c) A microtubule-depolymerizing drug, MBC, was added to a cell entering mitosis (0 min), right before SPB separation. MBC inhibited microtubule formation and SPB separation until the end of the observation (90 min). (d) MBC was added to a cell entering MII (n=14). Arrowheads indicate an SPB separation occurred even in the absence of ipMTs. (e) Time-lapse kymographs of the spindles during MII, without (left) and with (right) MBC (n≥10). The rectangle regions containing the spindles are cropped from the time-lapse images and aligned downward in the course of time. SPBs and kinetochores separated even in the absence of ipMTs (right). The length of the arrows corresponds to 5 min. (f) Nuclear division of MII zygotes without (left) and with (right) MBC was monitored with the nuclear envelope marker Cut11-3mRFP (red), together with GFP-Atb2 (green) (n≥6). The boxed regions are shown enlarged as time-lapse images below. (g)cut7-446mutant zygotes undergoing MII that were labelled with GFP-Atb2 (green), Mis6-2mRFP (red) and Sfi1-CFP (blue) (n=6). During MII, SPBs separated, and the bipolar spindle was formed at the restrictive temperature (32 °C), at which mitotic cells failed in SPB separation with the monopolar spindle. Scale bars, 2 μm. Figure 1: SPB separation with chromosome segregation and nuclear division occurred without interpolar microtubules (ipMTs) in meiosis II. ( a – e ) Live-cell imaging of cells carrying GFP-Atb2 (microtubules; green), Mis6-2mCherry (Mis6-2mCh; kinetochores; red) and Sfi1-CFP (SPBs; blue). Time-lapse images of cells undergoing normal mitosis ( a ) and meiosis II (MII) ( b ) are shown. For MII cells in b and d , the boxed regions of zygotes are shown enlarged as time-lapse images. The shape of cells is outlined in dotted curves; n =10. ( c ) A microtubule-depolymerizing drug, MBC, was added to a cell entering mitosis (0 min), right before SPB separation. MBC inhibited microtubule formation and SPB separation until the end of the observation (90 min). ( d ) MBC was added to a cell entering MII ( n =14). Arrowheads indicate an SPB separation occurred even in the absence of ipMTs. ( e ) Time-lapse kymographs of the spindles during MII, without (left) and with (right) MBC ( n ≥10). The rectangle regions containing the spindles are cropped from the time-lapse images and aligned downward in the course of time. SPBs and kinetochores separated even in the absence of ipMTs (right). The length of the arrows corresponds to 5 min. ( f ) Nuclear division of MII zygotes without (left) and with (right) MBC was monitored with the nuclear envelope marker Cut11-3mRFP (red), together with GFP-Atb2 (green) ( n ≥6). The boxed regions are shown enlarged as time-lapse images below. ( g ) cut7-446 mutant zygotes undergoing MII that were labelled with GFP-Atb2 (green), Mis6-2mRFP (red) and Sfi1-CFP (blue) ( n =6). During MII, SPBs separated, and the bipolar spindle was formed at the restrictive temperature (32 °C), at which mitotic cells failed in SPB separation with the monopolar spindle. Scale bars, 2 μm. Full size image Because it is possible that the effect of MBC was partial and that an undetectable amount of ipMTs remained and were able to carry out SPB separation and subsequent events, we then examined the cut7 mutant in our system. Cut7 is the fission yeast orthologue of the BimC/Eg5/kinesin-5 family kinesin [12] , [13] . Cut7 connects antiparallel microtubules that emanate from each SPB and slides the microtubules outward, thereby separating the SPBs. During mitosis, SPBs in the cut7-446 temperature-sensitive mutant failed to separate at the restrictive temperature, which resulted in the generation of monopolar spindles [13] ( Supplementary Fig. S2 ). In contrast, SPBs were able to separate during MII in cut7-446 zygotes at the restrictive temperature ( Fig. 1g ). This demonstrates that SPB separation during MII does not rely on the Cut7-mediated interaction of ipMTs. Thus, we conclude that ipMTs are dispensable in performing essential M-phase events, such as SPB separation, chromosome segregation and nuclear division in MII ( Supplementary Fig. S3 ). Normal chromosome segregation in absence of ipMTs in MII Mitotic cells treated with a high dose of MBC typically result in the lethal 'cut' phenotype, which displays enforced cytokinesis with unsegregated chromosomes [14] , [15] , [16] . To determine whether the ipMT-independent division observed during MII might result in abnormal segregation of chromosomes, we labelled the centromeres of chromosome II ( cen2 ) with GFP (the cen2 -GFP system [17] ) and filmed cells to make kymographs. During mitosis in the absence of MBC, a single Sfi1-CFP dot was split into two at the mitotic onset ( Supplementary Fig. S4a ). Simultaneously, the cen2 -GFP foci began to oscillate between the two SPBs until metaphase. The cen2 -GFP dots then separated towards each SPB (anaphase A), and the inter-SPB distance increased, reflecting spindle elongation (anaphase B) [17] , [18] . Similar kinetics was observed during MII (WT MII, –MBC, Fig. 2a ). When MBC was added at the mitotic onset, SPBs stopped splitting and the cen2 -GFP foci ceased oscillating ( Supplementary Fig. S4b ), resulting in a failure in chromosome segregation. In contrast, 80% of MII zygotes treated with MBC segregated cen2 -GFP to two poles (WT MII, +MBC, Fig. 2a,b ), indicating again that MII is much less sensitive to MBC than mitosis and MI. 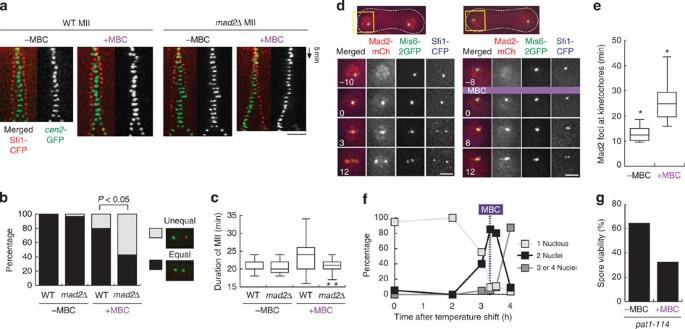Figure 2: Spindle-assembly checkpoint ensures chromosome segregation without interpolar microtubules during meiosis II. (a) Kymographs of wild-type (WT) andmad2Δ cells undergoing MII in the absence (−) or presence (+) of MBC (n≥14). Centromeres of chromosome II were labelled with GFP (cen2-GFP; green), and their SPBs were monitored with Sfi1-CFP (red). MBC was added before SPB separation. The length of arrows corresponds to 5 min. (b) The accuracy of chromosome segregation during MII in wild-type andmad2Δ cells was quantified (unpaired two-tailedt-test,n≥14). Typical images for equal and unequalcen2-GFP segregation are also shown. (c) The duration of MII was measured by monitoring the Cut11-3mRFP signals. Cut11-3mRFP formed foci at the SPBs at MII entry and disappeared at the onset of anaphase. Lines in the box-and-whisker plot from top to bottom are the maximum value, the 75th percentile, the median, the 25th percentile and the minimum value (n≥16). Asterisks indicate outliers. (d) Localization of Mad2 during MII in the absence (left) or presence (right) of MBC (n≥10). Mad2-mCherry (Mad2-mCh; red) was monitored with Mis6-2GFP (green) and Sfi1-CFP (blue). The time at which Mad2 foci first appeared at kinetochores is designated as 0 min. The addition of MBC retained Mad2 at kinetochores for >12 min, by which time Mad2 foci had translocated to SPBs in the absence of MBC. Scale bars, 2 μm. (e) The duration for Mad2 localization at kinetochores with or without MBC was determined from the observations ind. Note that Mad2-mCherry localization at SPBs, which means a release form the checkpoint activation, is not counted here. Lines in the box-and-whisker plot from top to bottom are the maximum value, the 75th percentile, the median, the 25th percentile and the minimum value (n≥10). Asterisks indicate outliers. (f) Meiotic progression of thepat1-114diploid synchronous culture was monitored by counting the number of nuclei per cell at each time point. Meiosis was induced by temperature shift (at 0 h). MBC was added when the population of binucleated (post-MI) cells was at a maximum (at 3.3 h). (g) Spore viability ofpat1-114diploid cells treated with or without MBC as infwas examined by tetrad analyses (n>300). Figure 2: Spindle-assembly checkpoint ensures chromosome segregation without interpolar microtubules during meiosis II. ( a ) Kymographs of wild-type (WT) and mad2 Δ cells undergoing MII in the absence (−) or presence (+) of MBC ( n ≥14). Centromeres of chromosome II were labelled with GFP ( cen2 -GFP; green), and their SPBs were monitored with Sfi1-CFP (red). MBC was added before SPB separation. The length of arrows corresponds to 5 min. ( b ) The accuracy of chromosome segregation during MII in wild-type and mad2 Δ cells was quantified (unpaired two-tailed t -test, n ≥14). Typical images for equal and unequal cen2 -GFP segregation are also shown. ( c ) The duration of MII was measured by monitoring the Cut11-3mRFP signals. Cut11-3mRFP formed foci at the SPBs at MII entry and disappeared at the onset of anaphase. Lines in the box-and-whisker plot from top to bottom are the maximum value, the 75th percentile, the median, the 25th percentile and the minimum value ( n ≥16). Asterisks indicate outliers. ( d ) Localization of Mad2 during MII in the absence (left) or presence (right) of MBC ( n ≥10). Mad2-mCherry (Mad2-mCh; red) was monitored with Mis6-2GFP (green) and Sfi1-CFP (blue). The time at which Mad2 foci first appeared at kinetochores is designated as 0 min. The addition of MBC retained Mad2 at kinetochores for >12 min, by which time Mad2 foci had translocated to SPBs in the absence of MBC. Scale bars, 2 μm. ( e ) The duration for Mad2 localization at kinetochores with or without MBC was determined from the observations in d . Note that Mad2-mCherry localization at SPBs, which means a release form the checkpoint activation, is not counted here. Lines in the box-and-whisker plot from top to bottom are the maximum value, the 75th percentile, the median, the 25th percentile and the minimum value ( n ≥10). Asterisks indicate outliers. ( f ) Meiotic progression of the pat1-114 diploid synchronous culture was monitored by counting the number of nuclei per cell at each time point. Meiosis was induced by temperature shift (at 0 h). MBC was added when the population of binucleated (post-MI) cells was at a maximum (at 3.3 h). ( g ) Spore viability of pat1-114 diploid cells treated with or without MBC as in f was examined by tetrad analyses ( n >300). Full size image In mitosis and MI, the spindle-assembly checkpoint (SAC) operates to monitor the attachment of microtubules to kinetochores. SAC components including Mad2 recognize unattached kinetochores and inhibit the activation of the anaphase-promoting complex/cyclosome so that cells can wait at metaphase until the attachment improves [19] . During mitosis, MBC causes spindle defects and activates SAC [15] , [20] . It is possible that SAC activity is required for the ipMT-independent MII caused by MBC. We thus monitored the behaviour of cen2 -GFP in the mad2 deletion ( mad2 Δ) mutant. In the absence of MBC, mad2 Δ zygotes underwent normal chromosome segregation as in wild-type zygotes ( mad2 Δ MII, –MBC, Fig. 2a,b ). When MBC was added at the onset of MII, ∼ 60% of mad2 Δ zygotes exhibited unequal segregation of cen2 -GFP, which was significantly higher than the ∼ 20% unequal segregation that occurred in wild-type zygotes ( Fig. 2b ). Wild-type zygotes treated with MBC during MII exhibited a delay in anaphase II onset ( Fig. 2c ). This was cancelled by removing Mad2, indicating that the delay was due to the SAC activation ( Fig. 2c ). In agreement with this, Mad2-mCherry showed prolonged localization to kinetochores in wild-type zygotes in the presence of MBC ( Fig. 2d,e ). These results indicate that, during MII in the presence of MBC, the proper attachment of microtubules to kinetochores is assured by Mad2-SAC, suggesting that the remnant short microtubules that survived after the MBC addition are indeed serving as ktMTs and that their proper attachment to kinetochores turns off the Mad2-SAC surveillance ( Supplementary Fig. S3e,f ). These results further indicate that the ipMT-independent division is unlikely to be a deregulated overrun that results in random chromosome segregation and tearing off the nucleus inappropriately like the lethal cut mutations. We next assessed whether MBC treatment during MII might affect spore viability. The pat1-114 mutant was used to induce synchronized meiosis [21] , [22] , [23] . MBC was added at 3.3 h after induction of meiosis, when the population of cells with two nuclei (meaning post-MI) was at a maximum ( ∼ 90%; Fig. 2f ). MBC caused a reduction in spore viability to 50% of that of the mock-treated cells ( Fig. 2g ). This value may reflect chromosome segregation fidelity: the frequency of faithful segregation of cen2 -GFP in MBC-treated MII cells was 80% ( Fig. 2b ), implying that the estimated frequency of equal segregation of all three chromosomes would be ∼ 51% ((0.8) 3 =0.512), which is comparable to the spore viability observed in the presence of MBC. The forespore membrane is responsible for MII without ipMTs Given that ipMTs were dispensable for the MII events, we wondered what might serve as the structural mainstay to separate SPBs and maintain the bipolar structure independently of ipMTs. As MII is coupled to sporulation (the terminal event in meiosis corresponding to gametogenesis in higher eukaryotes), we suspected that some sporulation-related cytoskeletal system might be involved in the ipMT-independent events. A candidate could be the forespore membrane, which is a precursor of the spore plasma membrane that surrounds nuclei during MII [24] . The forespore membrane was visualized with the GFP-tagged t-SNARE protein Psy1/Syntaxin 1 (GFP-Psy1) [25] . As reported previously [26] , the forespore membrane started to assemble around the SPBs in a crescent shape after they were separated by ipMTs (15 min; Fig. 3a ). The membrane gradually encapsulated the nuclei as anaphase II proceeded (36 min and 72 min). In MBC-treated zygotes, however, SPB separation without ipMTs occurred simultaneously with the initiation of forespore membrane growth (30–35 min; Fig. 3a ). The forespore membrane continued to grow and finally surrounded the two nuclei, resulting in their division (100 min). This led us to hypothesize that, in the absence of ipMTs, the forespore membrane may serve as a structural backbone, the outward growth of which could generate a force that separates SPBs and constricts the nucleus. 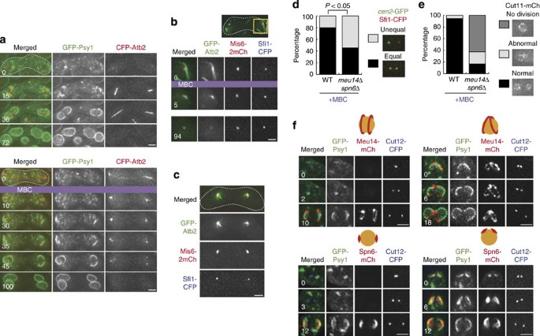Figure 3: The forespore membrane is responsible for meiosis II progression without interpolar microtubules. (a) Live-cell imaging of MII zygotes carrying GFP-Psy1 (forespore membrane; green) and CFP-Atb2 (red) in the absence of MBC (top) (n=18). MBC was added before the onset of MII (bottom) (n=18). SPB separation occurred concomitantly with initiation of the forespore membrane assembly. (b) MII ofspo15Δ cells carrying GFP-Atb2, Mis6-2mCherry (Mis6-2mCh) and Sfi1-CFP was filmed in the presence of MBC (n=10). SPBs had not separated by the end of the observation (94 min). (c) Thespo15Δcut7-446double mutant carrying GFP-Atb2, Mis6-2mCherry and Sfi1-CFP undergoing MII at the restrictive temperature. The double mutant exhibited the monopolar spindle phenotype (n=8), indicating that the forespore membrane has a crucial role in bipolar spindle formation during MII incut7-446cells. (d) Sister-chromatid segregation patterns during MII in wild-type andmeu14Δspn6Δ zygotes monitored bycen2-GFP with Sfi1-CFP (unpaired two-tailedt-test,n≥14). Typical images for equal and unequalcen2-GFP segregation are also shown. (e) Nuclear division during MII of wild-type andmeu14Δspn6Δ zygotes was monitored by Cut11-mCherry (Cut11-mCh); cells were categorized as undergoing normal division, abnormal division or no division (n≥18). Typical images for each category are also shown. (f) The leading edge ring formed above the nucleus was visualized with Meu14-mCherry (Meu14-mCh) (n≥24). (Top, left) In the absence of MBC, the leading edge rings were formed after SPB separation. (Top, right) In the presence of MBC, the leading edge rings formed from each SPB made contact with each other, which was maintained during SPB separation (indicated by an SPB marker, Cut12-CFP) and forespore membrane growth (visualized with GFP-Psy1). Schematic drawings for nuclei (orange) and leading edge rings (red) are also shown. (Bottom) The septin complex was visualized with Spn6-mCherry (Spn6-mCh) (n≥8). (Bottom left) In the absence of MBC. (Bottom right) In the presence of MBC. Drawings for nuclei (orange) and the septin complex (red) are also shown. Scale bars, 2 μm. Figure 3: The forespore membrane is responsible for meiosis II progression without interpolar microtubules. ( a ) Live-cell imaging of MII zygotes carrying GFP-Psy1 (forespore membrane; green) and CFP-Atb2 (red) in the absence of MBC (top) ( n =18). MBC was added before the onset of MII (bottom) ( n =18). SPB separation occurred concomitantly with initiation of the forespore membrane assembly. ( b ) MII of spo15 Δ cells carrying GFP-Atb2, Mis6-2mCherry (Mis6-2mCh) and Sfi1-CFP was filmed in the presence of MBC ( n =10). SPBs had not separated by the end of the observation (94 min). ( c ) The spo15 Δ cut7-446 double mutant carrying GFP-Atb2, Mis6-2mCherry and Sfi1-CFP undergoing MII at the restrictive temperature. The double mutant exhibited the monopolar spindle phenotype ( n =8), indicating that the forespore membrane has a crucial role in bipolar spindle formation during MII in cut7-446 cells. ( d ) Sister-chromatid segregation patterns during MII in wild-type and meu14 Δ spn6 Δ zygotes monitored by cen2 -GFP with Sfi1-CFP (unpaired two-tailed t -test, n ≥14). Typical images for equal and unequal cen2 -GFP segregation are also shown. ( e ) Nuclear division during MII of wild-type and meu14 Δ spn6 Δ zygotes was monitored by Cut11-mCherry (Cut11-mCh); cells were categorized as undergoing normal division, abnormal division or no division ( n ≥18). Typical images for each category are also shown. ( f ) The leading edge ring formed above the nucleus was visualized with Meu14-mCherry (Meu14-mCh) ( n ≥24). (Top, left) In the absence of MBC, the leading edge rings were formed after SPB separation. (Top, right) In the presence of MBC, the leading edge rings formed from each SPB made contact with each other, which was maintained during SPB separation (indicated by an SPB marker, Cut12-CFP) and forespore membrane growth (visualized with GFP-Psy1). Schematic drawings for nuclei (orange) and leading edge rings (red) are also shown. (Bottom) The septin complex was visualized with Spn6-mCherry (Spn6-mCh) ( n ≥8). (Bottom left) In the absence of MBC. (Bottom right) In the presence of MBC. Drawings for nuclei (orange) and the septin complex (red) are also shown. Scale bars, 2 μm. Full size image If the forespore membrane drives SPB separation in the absence of ipMTs, simultaneous inhibition of the forespore membrane and microtubule formation will hamper it. To test this possibility, we used the spo15 Δ mutant, in which SPBs are not properly modified and the forespore membrane does not assemble on them [27] . SPB separation was never observed in spo15 Δ cells treated with MBC (94 min; Fig. 3b ), demonstrating that it was indeed the forespore membrane that drove SPB separation in the absence of ipMTs. Moreover, neither chromosome segregation nor nuclear division was observed. Similarly, the SPB separation that took place during MII in cut7-446 zygotes was blocked by the spo15 deletion ( Fig. 3c ). Thus, the forespore membrane compensates for the structural defects of the bipolar spindle caused by a loss of ipMTs or a failure in the sliding of antiparallel microtubules. Both spo15 Δ cells treated with MBC ( Fig. 3b ) and spo15 Δ cut7-446 cells ( Fig. 3c ) failed to separate SPBs, segregate chromosomes and divide the nucleus, even though those cells had remnant microtubules around the SPBs. These observations demonstrate that those ipMT-independent meiotic events are controlled solely by the forespore membrane, but not by the remaining ktMTs. The leading edge ring and the septin complex The growing edge of the forespore membrane is fringed by the leading edge structure, which contains proteins such as Meu14 (refs 28 , 29 ) and is supported by the complex of septins [30] (Spn2, Spn5, Spn6 and Spn7). Both the leading-edge structure and the septin complex are required to navigate forespore membrane growth in the proper direction [30] . We blocked the function of both structures by using the meu14 Δ spn6 Δ double mutant to disorient the growth of the forespore membrane. MBC-treated meu14 Δ spn6 Δ cells could separate SPBs during MII to some extent, probably because the forespore membrane could initially assemble without septins and Meu14. These cells, however, frequently failed in segregating sister chromatids equally and in executing nuclear division ( Fig. 3d,e ). Significantly, leading edge rings formed from both SPBs made and kept physical contact with each other when the SPBs separated in the absence of ipMTs ( Fig. 3f ). The septin complex visualized by Spn6-mCherry also appeared simultaneously with the emergence of leading edge rings to align the forespore membrane ( Fig. 3f ). These results taken together provide genetic and visual evidence that the forespore membrane properly oriented by the leading edge ring generates an interpolar tension, which indeed leads to constant separation of SPBs, chromosome segregation and nuclear constriction. The leading edge ring containing Meu14 is backed with F-actin [31] . When actin polymerization was inhibited with latrunculin A in the presence of MBC, the leading edge ring did not constrict and failed in chromosome segregation and nuclear division, although SPB separation occurred ( Supplementary Fig. S5 ). This phenotype is similar to that of meu14 Δ spn6 Δ, validating the functional relationship of the leading edge ring and actin. Contribution of the forespore membrane to physiological MII All the results above suggest that the forespore membrane functions as a structural device that assists the spindle. To test whether the forespore-membrane-mediated machinery also contributes to physiological MII, in which microtubules are unperturbed, we used the spo15 Δ mutant, which does not form the forespore membrane. Although Spo15 is not essential for MII progression [27] , we particularly focused on the fidelity of SPB separation by monitoring a component of the nuclear pore complex, Cut11-3mRFP. This protein localizes to SPBs when they are embedded in the nuclear envelope at the onset of M-phase [32] ( Fig. 4a ) and are no longer associated with them at the onset of anaphase. For each nucleus, we recorded the timing of SPB separation as indicated by the split of the single Cut11-3mRFP focus. Remarkably, spo15 Δ cells during MII occasionally showed the disappearance of a single Cut11 dot without separation, suggesting that SPB separation did not occur in MII ( Fig. 4a and Table 1 ). No failure in SPB separation was observed during mitosis and MI in spo15 Δ cells ( Fig. 4a and Table 1 ). Thus, the forespore membrane, at least in part, contributes to efficient SPB separation during physiological MII. 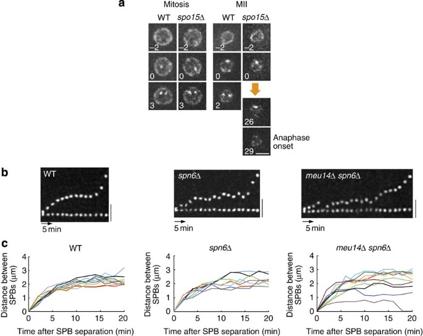Figure 4: The forespore membrane assists progression of physiological meiosis II. (a) Behaviour of Cut11-3mRFP was filmed in wild-type andspo15Δ cells at the onset of mitosis and MII (n≥26). In wild-type (WT) cells, Cut11-3mRFP constitutively localized to the nuclear envelope and additionally formed foci at the SPBs at mitotic/MII entry; this localization continued through SPB separation (visible as two foci) and disappeared at the onset of anaphase. Inspo15Δ cells at MII entry, however, Cut11-3mRFP foci occasionally disappeared without splitting, indicating a failure in SPB separation by the onset of anaphase (26–29 min). (b) Time-lapse kymographs showing the kinetics of the spindle during MII in wild-type,spn6Δ andmeu14Δspn6Δ cells (n≥8). One of the two Cut12-CFP dots (SPBs) at each time point was aligned at the bottom of the image to clarify an increment of the inter-SPB distance. The length of arrows corresponds to 5 min. Scale bars, 2 μm. (c) The kinetics of the SPBs in wild-type,spn6Δ andmeu14Δspn6Δ cells observed inbwere plotted. Each line represents the kinetics for a single nucleus (n≥8). Figure 4: The forespore membrane assists progression of physiological meiosis II. ( a ) Behaviour of Cut11-3mRFP was filmed in wild-type and spo15 Δ cells at the onset of mitosis and MII ( n ≥26). In wild-type (WT) cells, Cut11-3mRFP constitutively localized to the nuclear envelope and additionally formed foci at the SPBs at mitotic/MII entry; this localization continued through SPB separation (visible as two foci) and disappeared at the onset of anaphase. In spo15 Δ cells at MII entry, however, Cut11-3mRFP foci occasionally disappeared without splitting, indicating a failure in SPB separation by the onset of anaphase (26–29 min). ( b ) Time-lapse kymographs showing the kinetics of the spindle during MII in wild-type, spn6 Δ and meu14 Δ spn6 Δ cells ( n ≥8). One of the two Cut12-CFP dots (SPBs) at each time point was aligned at the bottom of the image to clarify an increment of the inter-SPB distance. The length of arrows corresponds to 5 min. Scale bars, 2 μm. ( c ) The kinetics of the SPBs in wild-type, spn6 Δ and meu14 Δ spn6 Δ cells observed in b were plotted. Each line represents the kinetics for a single nucleus ( n ≥8). Full size image Table 1 Frequency of cells showing a failure in SPB separation in mitosis and meiosis. Full size table To further investigate whether forespore membrane growth contributes to SPB separation during physiological MII, we monitored the kinetics of the inter-SPB distance (marked by Cut12-CFP). The inter-SPB distance increased over time in a stepwise manner during MII in wild-type cells, as occurred during mitosis ( Fig. 4b,c ). In contrast, disoriented growth of the forespore membrane in meu14 Δ spn6 Δ cells was frequently associated with a fluctuation in the inter-SPB distance ( Fig. 4b,c ). A similar but less remarkable fluctuation was seen in the spn6 Δ single mutant ( Fig. 4b,c ), indicating that Meu14 and Spn6 function in the forespore membrane guidance in a parallel pathway [30] ( Fig. 5a for a schematic). The velocity of SPB separation in meu14 Δ spn6 Δ cells could be transiently faster than that in wild-type cells ( Fig. 4c ), probably because the disoriented growth of the forespore membrane in them accordingly enforced a rapid separation of the SPBs. These results demonstrate that the dynamics of the forespore membrane indeed contribute to the kinetics of SPB separation during MII under physiological conditions. Moreover, meu14 Δ spn6 Δ cells showed abnormal division in as many as 20% of MII nuclei, suggesting the importance of the proper forespore membrane organization for accurate constriction of the nucleus. 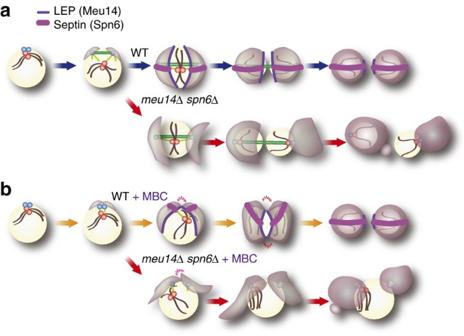Figure 5: Schematic illustration of forespore-membrane-mediated meiosis II. (a) Schematic illustration of the function of septins and leading-edge proteins (LEPs) in forespore membrane assembly. Septins and LEPs have important roles in forespore membrane orientation. In the wild type (WT), the growing edge of the forespore membrane is fringed by LEPs including Meu14 to properly orient and constrict the forespore membrane. The meiotic septin complex (Spn2, Spn5, Spn6 and Spn7) orients the growing direction of the edge. Septins and LEPs cooperatively control the direction of the growth of the forespore membrane. The sporulation-deficient phenotype is most prominent whenspn6Δ is combined withmeu14Δ; therefore, themeu14Δspn6Δ double mutant was used in this study as a strain that lacks both septins and LEPs. Inmeu14Δspn6Δ cells, the forespore membrane cannot encapsulate the nucleus properly, leading to production of defective spores. (b) This study proposes a novel role for septins and LEPs in chromosome segregation and nuclear division during MII. In the absence of ipMTs (WT+MBC), the forespore membrane, which begins to assemble from the SPBs, splits the SPBs. The forespore membrane is then guided by structures containing septins and LEPs to surround the nucleus. When MBC is added tomeu14Δspn6Δ cells (meu14Δspn6Δ+MBC), the forespore membrane assembly is disoriented, and neither chromosome segregation nor nuclear division takes place. As the microtubule-emanating SPBs are connected to the forespore membrane, its uncoordinated assembly may affect the efficiency and fidelity of kinetochore-microtubule attachment. Furthermore, septins and LEPs constrict the ipMT-free nucleus by generating a force that is normally used to encapsulate the nucleus after the ipMT-mediated nuclear division in wild-type MII. Figure 5: Schematic illustration of forespore-membrane-mediated meiosis II. ( a ) Schematic illustration of the function of septins and leading-edge proteins (LEPs) in forespore membrane assembly. Septins and LEPs have important roles in forespore membrane orientation. In the wild type (WT), the growing edge of the forespore membrane is fringed by LEPs including Meu14 to properly orient and constrict the forespore membrane. The meiotic septin complex (Spn2, Spn5, Spn6 and Spn7) orients the growing direction of the edge. Septins and LEPs cooperatively control the direction of the growth of the forespore membrane. The sporulation-deficient phenotype is most prominent when spn6 Δ is combined with meu14 Δ; therefore, the meu14 Δ spn6 Δ double mutant was used in this study as a strain that lacks both septins and LEPs. In meu14 Δ spn6 Δ cells, the forespore membrane cannot encapsulate the nucleus properly, leading to production of defective spores. ( b ) This study proposes a novel role for septins and LEPs in chromosome segregation and nuclear division during MII. In the absence of ipMTs (WT+MBC), the forespore membrane, which begins to assemble from the SPBs, splits the SPBs. The forespore membrane is then guided by structures containing septins and LEPs to surround the nucleus. When MBC is added to meu14 Δ spn6 Δ cells ( meu14 Δ spn6 Δ+MBC), the forespore membrane assembly is disoriented, and neither chromosome segregation nor nuclear division takes place. As the microtubule-emanating SPBs are connected to the forespore membrane, its uncoordinated assembly may affect the efficiency and fidelity of kinetochore-microtubule attachment. Furthermore, septins and LEPs constrict the ipMT-free nucleus by generating a force that is normally used to encapsulate the nucleus after the ipMT-mediated nuclear division in wild-type MII. Full size image We have demonstrated the unprecedented function of the forespore membrane in SPB separation, chromosome segregation and nuclear division during MII. We propose that, at the initial stage of MII, the developing forespore membrane generates SPB-separating force from the paired SPBs outward along the nuclear membrane, and then supports the bipolar spindle for efficient chromosome segregation. In the absence of ipMTs, the leading edge structures developed from the two SPBs collide, and their repulsive force generates a physical tension between the SPBs ( Fig. 5 ). The forespore-membrane-mediated division apparatus, reinforced by the leading edge structure and septins, may facilitate the equal segregation of chromosomes and constriction of the nuclear envelope, even in the absence of ipMTs. Interestingly, Mad2-SAC was required to ensure the proper timing of chromosome segregation in the absence of ipMTs, implying that forespore-membrane-mediated nuclear constriction could be regulated by the anaphase-promoting complex/cyclosome. Based on the ability of the forespore membrane to compensate for the absence of ipMTs during MII, we believe that the crucial functions of ipMTs are as follows: to anchor spindle poles to the nuclear envelope to secure fulcra for the force of chromosome segregation and to divide the nucleus in anaphase. Cell division without the tubulin homologue FtsZ occurs in strains of the bacterium Bacillus subtilis that are defective in cell wall organization [33] . It has been reported recently that a microtubule-independent nuclear division (nuclear fission) occurs in S. pombe mitosis when cytokinesis (cell wall formation at mitotic exit) is artificially inhibited [16] , although how the force is generated remains unclear. In this study we have clarified the mechanics to generate the force necessary for nuclear division without ipMTs during MII: the physical contact of forespore membrane edges is the pivot. In contrast to the previous studies for mitosis, the forespore-membrane-mediated force apparently contributes to physiological MII. We speculate that such forespore-membrane-mediated machinery may have developed as a backup system for chromosome segregation during MII, in which the spindle structure may not be as robust as it is during mitosis or MI. The meiotic spindle is first built during MI and then disassembled, followed by the reconstruction during MII. Notably, MII is a 'virtually open-meiosis' in which nuclear proteins disperse out of the nucleus during anaphase [34] , [35] . These situations may imply that the spindle organization could be less efficient in MII than in mitosis. Moreover, MII should couple with encapsulation of sister nuclei by forespore membrane. The forespore membrane therefore may have necessitated the ability to generate a force that assists the functions of the spindle. The membrane structure involving leading-edge proteins and septins thus has acquired a dual function: encapsulation of the nucleus and assistance of chromosome segregation. It is intriguing to note similarities and differences between this structure and the spindle matrix, which is supposed to maintain the spindle structure in higher eukaryotes, as a backbone made of non-microtubule materials [36] . A membranous organization that includes lamin B has been shown recently to function as a spindle matrix that surrounds the whole prometaphase spindle to maintain its structure [37] , [38] , [39] . In addition to being a structural scaffold, however, the forespore membrane can generate a force for SPB separation and nuclear division. Higher eukaryotes may have developed microtubule-dependent machinery as the advantageous force-generating device, and the membranous spindle matrix may have differentiated as a supporting structure. Yeast strains and genetic procedures Strains used in this study are listed in Supplementary Table S1 . The PCR-based standard methods for gene targeting [4] , [40] were used to construct gene disruptants and fluorescent protein-tagged strains with selection marker gene cassettes, except for the GFP-Psy1 strain [26] , which was constructed through integration of a plasmid that contains the GFP-Psy1 fusion construct (a gift from T. Nakamura). The cen2 -GFP strain was provided by A. Yamamoto [17] . Briefly, repetitive LacO sequences were inserted close to the centromere region of chromosome II ( cen2 ), which was recognized by a co-expressed LacI–nuclear localization signal–GFP fusion protein. For induction of meiosis, homothallic h 90 cells were spotted on the sporulation agar medium for all experiments except for the spore viability test shown in Fig. 2f,g (see below). Synchronization of meiosis and spore viability test For spore viability test ( Fig. 2f,g ), we used a system to induce synchronized meiosis using the diploid ( h − / h − ) pat1-114 + mat-Pc strain [41] , thereby determining when the binucleate population was at its peak (and thus when to add MBC). To monitor meiotic progression with the number of nuclei, cells were stained with 4′,6-diamino-2-phenylindole after being fixed in 50% methanol. Spore viability was examined by tetrad analyses. Spores were germinated on the rich yeast extract medium. The viability is the average of three independent experiments. Microscopy For live-cell imaging of mitotic cells, logarithmically growing cells cultured in the thiamine-rich synthetic defined medium at 30 °C for ≥13 h were used. For live-cell imaging of cells in meiosis, zygotes spotted on the sporulation agar medium at 25 °C for ≥8 h were used. Living cells were observed in Edinburgh minimal medium with or without a nitrogen source to analyse the mitotic cycle or meiosis, respectively. Live-cell imaging was performed as described [4] on a DeltaVision-SoftWoRx system (Applied Precision) using a microscope (IX71, Olympus) equipped with fluorescein isothiocyanate, mCherry and CFP filters (Chroma technology), a Plan Apo N ×60 (NA, 1.42) or a UPlan SApo ×100 (NA, 1.40) oil immersion objective lens (Olympus), a CoolSNAP HQ2 camera (Photometrics) and a temperature controller (Precision Control) at 25 °C, except for Figs 1g and 3c and Supplementary Figs S2 and S3e,f (32 °C was used for the cut7-446 and nuf2-1 temperature-sensitive mutant). z -Sectioning was carried out at 0.4- or 0.5-μm interval, and images were taken every 1 to 5 min. Images were then deconvolved, and a z -stack projection was created with the maximum or the sum method. The temperature shift for the temperature-sensitive mutants was performed at least 1 h before the observation. Drug treatment In live-cell imaging, images for the first time point were taken without MBC. MBC (Sigma-Aldrich) was then added at a final concentration of 50 μg ml −1 in all experiments. Latrunculin A (Invitrogen) was added at a final concentration of 50 μM at least 1 h before the live-cell imaging. Statistics An unpaired two-tailed t -test was used for statistical analyses. How to cite this article: Akera, T. et al . Interpolar microtubules are dispensable in fission yeast meiosis II. Nat. Commun. 3:695 doi: 10.1038/ncomms1725 (2012).